FoxO proteins restrain osteoclastogenesis and bone resorption by attenuating H2O2accumulation Besides their cell-damaging effects in the setting of oxidative stress, reactive oxygen species (ROS) play an important role in physiological intracellular signalling by triggering proliferation and survival. FoxO transcription factors counteract ROS generation by upregulating antioxidant enzymes. Here we show that intracellular H 2 O 2 accumulation is a critical and purposeful adaptation for the differentiation and survival of osteoclasts, the bone cells responsible for the resorption of mineralized bone matrix. Using mice with conditional loss or gain of FoxO transcription factor function, or mitochondria-targeted catalase in osteoclasts, we demonstrate this is achieved, at least in part, by downregulating the H 2 O 2 -inactivating enzyme catalase. Catalase downregulation results from the repression of the transcriptional activity of FoxO1, 3 and 4 by RANKL, the indispensable signal for the generation of osteoclasts, via an Akt-mediated mechanism. Notably, mitochondria-targeted catalase prevented the loss of bone caused by loss of oestrogens, suggesting that decreasing H 2 O 2 production in mitochondria may represent a rational pharmacotherapeutic approach to diseases with increased bone resorption. Resorption of the mineralized bone matrix—a physiologic process essential for skeletal and mineral homoeostasis—is the function of osteoclasts, giant multinucleated cells that are derived from myeloid lineage precursors [1] . Abnormal osteoclast generation and/or lifespan is responsible for many of the benign or malignant diseases of bone, including postmenopausal osteoporosis [2] , [3] . During osteoclastogenesis, bone marrow macrophages (BMMs) differentiate into tartrate-resistant acid phosphatase (TRAP)-positive pre-osteoclasts, which then fuse with each other to form mature osteoclasts. These highly specialized cells are uniquely capable of dissolving and digesting the organic bone matrix by virtue of their ability to secrete protons and lysosomal enzymes into a sealed microenvironment formed by a ‘podosome belt’ that tightly adheres to the bone area targeted for removal [4] , [5] , [6] . Macrophage colony-stimulating factor (M-CSF) and receptor activator of nuclear factor-B ligand (RANKL) provide the two necessary and sufficient signals for osteoclast differentiation. Binding of M-CSF to its receptor CSF-1R in osteoclast precursors promotes their proliferation and survival via the activation of kinases such as Src, PLC-γ, PI(3)K, Akt and Erk [7] , [8] , [9] . RANKL binding to RANK induces the association of RANK with TRAF6, which activates NF-kB and MAPKs (Erk, JNK and p38). These kinases, in turn, activate NFATc1, the master transcription factor responsible for osteoclast differentiation and function [10] . Over 20 years ago, results of experiments with organ cultures, showing that osteoclast formation in response to parathyroid hormone and interleukin-1 is associated with superoxide anion generation and that superoxide dismutase attenuates osteoclastic resorption, suggested that reactive oxygen species (ROS) play a role in osteoclast differentiation and bone resorption [11] . Subsequent in vitro work has shown that both RANKL and M-CSF increase the levels of ROS in osteoclast progenitors and that the increase in ROS may potentiate osteoclast formation, activation and survival [12] , [13] , [14] . In addition, an increase in osteoclast ROS has been associated with mitochondria biogenesis orchestrated by PGC-1β in mice [15] . An increase in the generation of ROS has been also implicated in the pathologic bone resorption associated with oestrogen deficiency and inflammatory arthritis [16] , [17] , [18] . However, in all of these previous studies, the link between ROS generation and osteoclast formation has been circumstantial. Specifically, heretofore, there has been no direct evidence that ROS production in osteoclasts or their progenitors is important for osteoclastogenesis in vivo or skeletal homoeostasis. Moreover, there has been no mechanistic explanation for how oxygen radicals increase during osteoclast differentiation, either in vitro or in vivo . Several antioxidant enzymes, including peroxiredoxins, glutathione peroxidases and catalase, prevent H 2 O 2 accumulation and cell damage [19] . In some cell types—for example, haematopoietic stem cells—the forkhead box O (FoxO) family of transcription factors reduce ROS by upregulating the expression of antioxidant enzymes [20] , [21] . Mammalian FoxO1, 3 and 4 are negatively regulated by insulin and growth factors via the serine/threonine kinase Akt [22] . Akt directly phosphorylates FoxOs and this results in their retention in the cytoplasm and thereby abrogation of FoxO-mediated transcription. In contrast, stress stimuli such as growth factor depletion or oxidative stress leads to the retention of FoxOs in the nucleus and activation of transcription of genes involved in cell cycle arrest, differentiation, apoptosis, autophagy, metabolism and stress resistance. Earlier work by us and others has established that FoxOs play an important role in bone metabolism by influencing osteoblast generation and survival via ROS-dependent and -independent mechanisms [23] , [24] , [25] . Nonetheless, FoxO1, 3 and 4 are also expressed in cells of the haematopoietic lineage [20] , [26] , and global combined deletion of FoxO1, 3 and 4 in our earlier work increased the number of osteoclast progenitors in the bone marrow [23] . However, it remains unknown whether FoxOs have a cell-autonomous effect in cells of the osteoclast lineage. The work reported herein reveals that FoxOs do indeed have a cell-autonomous effect in osteoclasts. Specifically, using mice with conditional loss or gain of FoxO function or mitochondria-targeted catalase in osteoclasts we show that M-CSF- and RANKL-induced Akt activation downregulates FoxOs, thereby decreasing catalase and allowing the accumulation of H 2 O 2 . This cascade of events is a critical control node of osteoclastogenesis and bone resorption, under both physiologic and pathologic conditions. RANKL decreases FoxO transcriptional activity in osteoclasts FoxO1, 3 and 4 mRNA and protein levels were greatly decreased during the transition of BMMs to mature osteoclasts in the presence of RANKL ( Fig. 1a,b ). A detailed time course, following the addition of RANKL, elucidated that the decrease in FoxO protein levels occurred as early as 3 h ( Supplementary Fig. 1 ). RANKL also attenuated FoxO-mediated transcription dose-dependently in Raw264.7 macrophages transfected with a FoxO-luc reporter construct ( Fig. 1c ). The suppressive effect of RANKL on FoxO-luc activity in Raw264.7 cells was present even in the absence of serum, which is a strong stimulus for FoxO-mediated transcription [27] . Moreover, RANKL attenuated FoxO-luc activity in Raw264.7 cells in which FoxO1, FoxO3 or FoxO4 expression levels were increased by transfection of the respective plasmids ( Fig. 1d ), indicating that RANKL has a similar effect on the function of all three proteins. To confirm the suppressive effect of RANKL on FoxO transcriptional activity by alternative means, we examined the nuclear localization of FoxOs in BMMs. Serum deprivation promoted FoxO1, FoxO3 or FoxO4 accumulation in the nucleus, whereas RANKL decreased the nuclear levels of FoxOs independent of the presence or absence of serum ( Fig. 1e ). In agreement with the inhibitory effect of RANKL on FoxO-mediated transcription, the expression of the FoxO target gene catalase [28] was decreased in pre-osteoclasts and mature osteoclasts as compared with BMMs ( Fig. 1f ). 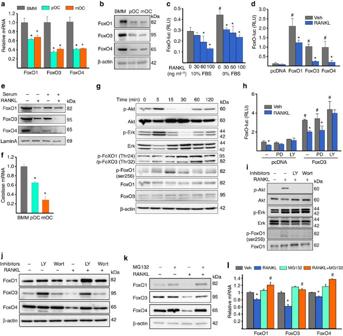Figure 1: RANKL decreases FoxO levels and activity. (a) FoxO mRNA (triplicates) and (b) protein levels in BMMs, pre-osteoclasts (pOC) and mature (m) osteoclast cultures. (c) Luciferase activity in RAW264.7 cells transfected with a FoxO-luc reporter construct and incubated with the indicated doses of RANKL in the presence or absence of fetal bovine serum (FBS) for 16 h (triplicates). RLU, relative luminescence units. *P<0.05 versus respective untreated cells,#P<0.05 versus untreated cells in 10% serum. (d) Luciferase activity as incin cells co-transfected with a control plasmid (pcDNA) or with plasmids expressing FoxO1, 3 or 4 and treated with 60 ng ml−1RANKL. *P<0.05 versus respective vehicle (veh)-treated cells,#P<0.05 versus veh-treated cells with pcDNA. (e) Protein levels of FoxOs and the nuclear protein lamin A in nuclear extract of BMMs incubated with or without RANKL in the absence or presence of 10% FBS. (f) Catalase mRNA levels in cells described ina. *P<0.05. (g) RANKL-induced Akt, Erk, FoxO1 and FoxO3 phosphorylation in BMMs. (h) Luciferase activity as indin cells treated with veh, 50 nM PD98059 and 10 μM LY294002. *P<0.05 versus respective veh-treated cells,#P<0.05 versus similar treated cells with pcDNA. (i) Akt, Erk and FoxO1 phosphorylation in BMMs induced by RANKL for 15 min in the presence or absence of 10 μM LY294002 or 0.2 μM wortmannin. (j) Protein levels of FoxOs in cells treated similar to that inifor 2 days. (k,l) BMM incubated with or without RANKL for 6 h (k) or 3 h (l) in the presence or absence of 20 mM MG132. *P<0.05 versus respective veh-treated cells,#P<0.05 versus RANKL alone. Bars represent mean and s.d.; Student’st-test. Figure 1: RANKL decreases FoxO levels and activity. ( a ) FoxO mRNA (triplicates) and ( b ) protein levels in BMMs, pre-osteoclasts (pOC) and mature (m) osteoclast cultures. ( c ) Luciferase activity in RAW264.7 cells transfected with a FoxO-luc reporter construct and incubated with the indicated doses of RANKL in the presence or absence of fetal bovine serum (FBS) for 16 h (triplicates). RLU, relative luminescence units. * P <0.05 versus respective untreated cells, # P <0.05 versus untreated cells in 10% serum. ( d ) Luciferase activity as in c in cells co-transfected with a control plasmid (pcDNA) or with plasmids expressing FoxO1, 3 or 4 and treated with 60 ng ml −1 RANKL. * P <0.05 versus respective vehicle (veh)-treated cells, # P <0.05 versus veh-treated cells with pcDNA. ( e ) Protein levels of FoxOs and the nuclear protein lamin A in nuclear extract of BMMs incubated with or without RANKL in the absence or presence of 10% FBS. ( f ) Catalase mRNA levels in cells described in a . * P <0.05. ( g ) RANKL-induced Akt, Erk, FoxO1 and FoxO3 phosphorylation in BMMs. ( h ) Luciferase activity as in d in cells treated with veh, 50 nM PD98059 and 10 μM LY294002. * P <0.05 versus respective veh-treated cells, # P <0.05 versus similar treated cells with pcDNA. ( i ) Akt, Erk and FoxO1 phosphorylation in BMMs induced by RANKL for 15 min in the presence or absence of 10 μM LY294002 or 0.2 μM wortmannin. ( j ) Protein levels of FoxOs in cells treated similar to that in i for 2 days. ( k , l ) BMM incubated with or without RANKL for 6 h ( k ) or 3 h ( l ) in the presence or absence of 20 mM MG132. * P <0.05 versus respective veh-treated cells, # P <0.05 versus RANKL alone. Bars represent mean and s.d. ; Student’s t -test. Full size image RANKL activates Akt and Erk, which, in turn, decrease FoxO activity by increasing FoxO phosphorylation [27] , [29] . In line with this evidence, the RANKL-induced increase in the phosphorylation of Akt and Erk preceded the phosphorylation of FoxO1 and FoxO3 in BMMs ( Fig. 1g ). Moreover, the attenuating effect of RANKL on FoxO-luc activity was prevented by LY294002, an inhibitor of PI3K/Akt, but not by PD98059, an inhibitor of Erk ( Fig. 1h ), indicating that Akt mediated the effects of RANKL on FoxO activity. In agreement with this contention, the phosphorylation of FoxO1 by RANKL was abrogated by LY294002 or wortmannin, another inhibitor of PI3K/Akt ( Fig. 1i ). Similarly, these two inhibitors prevented the RANKL-induced decrease in FoxO1, FoxO3 and FoxO4 protein levels ( Fig. 1j ). Akt phosphorylation can cause proteasomal degradation of FoxOs [30] . Using the proteasome inhibitor MG132, we determined that the RANKL-induced decrease of FoxOs resulted from proteasomal degradation ( Fig. 1k ). FoxOs can self-amplify at least in some cell types [31] , raising the possibility that a decrease in FoxO protein levels might decrease the transcription of the FoxO genes. In line with this, we found that the decline in FoxO1, 3 and 4 mRNA levels, seen as early as 3 h following addition of RANKL, was also prevented by MG132 ( Fig. 1l ). The results of this section, taken together with the published evidence, indicate that RANKL decreases both the transcriptional activity and the protein levels of FoxOs in osteoclast progenitors via Akt stimulation. Deletion of FoxOs in osteoclasts decreases bone mass We next deleted FoxO1 , FoxO3 and FoxO4 in osteoclast precursors in mice by crossing floxed FoxO1, 3 and 4 mice (FoxO1,3,4 f/f ) with LysM-Cre mice, in which the Cre recombinase is expressed in cells of the monocyte/macrophage lineage and neutrophils [32] . Mice lacking FoxO1, 3 and 4 in LysM-Cre-expressing cells, hereafter referred to as FoxO1,3,4 f/f ;LysM-Cre mice, were born at the expected Mendelian ratio and their body weight was indistinguishable from control FoxO1,3,4 f/f littermates ( Supplementary Fig. 2a ). FoxO1, 3 and 4 mRNA levels were reduced by ~80% in macrophages from FoxO1,3,4 f/f ;LysM-Cre mice cultured in the presence of M-CSF ( Fig. 2a ). The mRNA and protein levels of FoxOs were also decreased in osteoclasts cultured in the presence of RANKL ( Fig. 2b ). FoxO mRNA was unaltered in bone marrow-derived osteoblastic cells from FoxO1,3,4 f/f ; LysM-Cre mice, demonstrating the specificity of the deletion ( Supplementary Fig. 2b ). 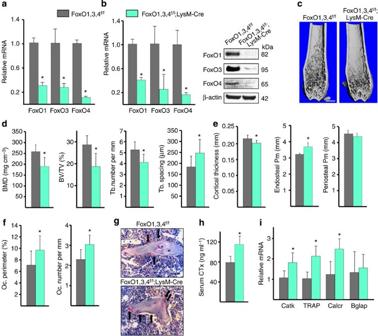Figure 2: Deletion of FoxOs in osteoclasts increases bone resorption. (a) FoxOs mRNA levels in BMM cultures (triplicates). (b) FoxOs mRNA (right) and protein (left) in mature osteoclast cultures. (c) Representative μCT images of distal femur of 6-week-old male mice. Scale bar, 1 mm. (d) Cancellous BMD, bone volume relative to the total volume (BV/TV) and trabecular (Tb) number, thickness and spacing in distal femur of 6-week-old male FoxO1,3,4f/f(n=10) and FoxO1,3,4f/f;LysM-Cre (n=8) littermates. (e) Cortical bone measurements determined using micro-CT in femoral diaphysis of the samples described ind. Pm, perimeter. (f) Osteoclasts in cancellous bone of vertebra from FoxO1,3,4f/f(n=8) and FoxO1,3,4f/f;LysM-Cre (n=11) mice described ind. (g) Histological sections of bone, described inf, stained for TRAP activity (osteoclasts stain red). Scale bar, 20 μm. (h) Serum concentration of a collagen degradation product (CTx) in mice described ind(n=8 mice per group). (i) Cathepsin K (CatK), TRAP, calcitonin receptor (calcr) and osteocalcin (OCN) mRNA levels in vertebrae of mice described ind(n=6 mice per group). Bars represent mean and s.d. *P<0.05 versus FoxO1,3,4f/fby Student’st-test. Figure 2: Deletion of FoxOs in osteoclasts increases bone resorption. ( a ) FoxOs mRNA levels in BMM cultures (triplicates). ( b ) FoxOs mRNA (right) and protein (left) in mature osteoclast cultures. ( c ) Representative μCT images of distal femur of 6-week-old male mice. Scale bar, 1 mm. ( d ) Cancellous BMD, bone volume relative to the total volume (BV/TV) and trabecular (Tb) number, thickness and spacing in distal femur of 6-week-old male FoxO1,3,4 f/f ( n =10) and FoxO1,3,4 f/f ;LysM-Cre ( n =8) littermates. ( e ) Cortical bone measurements determined using micro-CT in femoral diaphysis of the samples described in d . Pm, perimeter. ( f ) Osteoclasts in cancellous bone of vertebra from FoxO1,3,4 f/f ( n =8) and FoxO1,3,4 f/f ;LysM-Cre ( n =11) mice described in d . ( g ) Histological sections of bone, described in f , stained for TRAP activity (osteoclasts stain red). Scale bar, 20 μm. ( h ) Serum concentration of a collagen degradation product (CTx) in mice described in d ( n =8 mice per group). ( i ) Cathepsin K (CatK), TRAP, calcitonin receptor (calcr) and osteocalcin (OCN) mRNA levels in vertebrae of mice described in d ( n =6 mice per group). Bars represent mean and s.d. * P <0.05 versus FoxO1,3,4 f/f by Student’s t -test. Full size image FoxO1,3,4 f/f ;LysM-Cre mice exhibited decreased femoral cancellous bone mineral density (BMD) and bone volume at 6 ( Fig. 2c,d ) and 32 weeks of age ( Supplementary Table 1 ), as measured using micro-CT. These changes were associated with a decrease in trabecular number and an increase in trabecular spacing. FoxO1,3,4 f/f ;LysM-Cre mice also exhibited decreased cortical thickness ( Fig. 2e , Supplementary Table 1 ). This latter change resulted from an enlargement of the inner perimeter, indicative of increased endosteal resorption. Similar changes in cancellous bone were confirmed in the vertebrae of the FoxO1,3,4 f/f ;LysM-Cre mice ( Supplementary Fig. 3 , Supplementary Table 1 ). Histomorphometric analysis of the vertebrae from FoxO1,3,4 f/f ; LysM-Cre mice revealed that osteoclast number and perimeter were increased ( Fig. 2f,g ). The serum marker of bone resorption (CTx) was also increased in the FoxO1,3,4 f/f ;LysM-Cre mice ( Fig. 2h ), as was the expression of the osteoclast-specific markers cathepsin K (catk ), TRAP and calcitonin receptor ( calr ) in the bone ( Fig. 2i ). In contrast, the mRNA for the bone formation marker osteocalcin ( bglap ) was unaffected. FoxO3 overexpression in osteoclasts increases bone mass To verify the role of FoxOs in osteoclastogenesis in mice, we overexpressed FoxO3 in cells of the osteoclast lineage. This was accomplished by crossing mice with a conditionally activated wild-type FoxO3 transgene ( FoxO3 C ) [23] with LysM-Cre mice. The FoxO3 C transgene was highly expressed in calvaria, vertebra ( Supplementary Fig. 4a ) and cultured osteoclasts from FoxO3 C ;LysM-Cre mice ( Fig. 3a ); however, it was undetectable in the bone and osteoclasts from littermate controls harbouring the LysM-Cre transgene alone. Osteoclasts from FoxO3 C ;LysM-Cre mice exhibited twofold higher protein level of FoxO3 as compared with cells from control mice ( Fig. 3b ). We have previously documented that the insertion site of the FoxO3 C transgene has no effect on bone mass because mice carrying the FoxO3 C transgene without Cre activation have bone mass and architecture similar to wild-type littermates [23] . 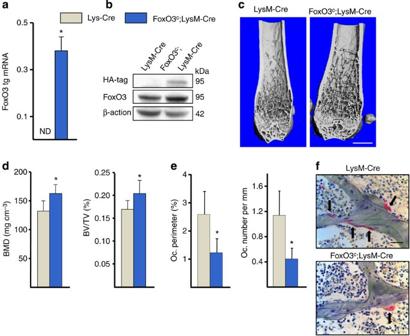Figure 3: Overexpression of FoxO3 in osteoclasts decreases bone resorption. (a) FoxO3 transgene mRNA and (b) protein in mature osteoclast cultures (triplicates); ND, not detected. (c) Representative μCT images of distal femur of 12-week-old male mice. Scale bar, 1 mm. (d) Cancellous BMD and bone volume relative to the total volume (BV/TV) of 12-week-old male LysM-Cre (n=12) and FoxO3C;LysM-Cre (n=13) littermates. (e) Osteoclasts in cancellous bone of vertebra from mice described ind(n=6 mice per group). (f) Histological sections of bone, described ine, stained for TRAP activity (osteoclasts stain red). Scale bar, 20 μm. Bars represent mean and s.d. *P<0.05 by Student’st-test. Figure 3: Overexpression of FoxO3 in osteoclasts decreases bone resorption. ( a ) FoxO3 transgene mRNA and ( b ) protein in mature osteoclast cultures (triplicates); ND, not detected. ( c ) Representative μCT images of distal femur of 12-week-old male mice. Scale bar, 1 mm. ( d ) Cancellous BMD and bone volume relative to the total volume (BV/TV) of 12-week-old male LysM-Cre ( n =12) and FoxO3 C ;LysM-Cre ( n =13) littermates. ( e ) Osteoclasts in cancellous bone of vertebra from mice described in d ( n =6 mice per group). ( f ) Histological sections of bone, described in e , stained for TRAP activity (osteoclasts stain red). Scale bar, 20 μm. Bars represent mean and s.d. * P <0.05 by Student’s t -test. Full size image Overexpression of FoxO3 in osteoclasts led to a significant increase in cancellous BMD and bone volume in the femurs of 12- ( Fig. 3c,d ) and 48-week-old mice ( Supplementary Table 2 ). These changes were accompanied by increased trabecular number and thickness, while trabecular spacing was decreased ( Supplementary Table 2 ). Similar changes were seen in vertebrae ( Supplementary Table 2 ). Cortical bone mass was also increased in FoxO3 C ;LysM-Cre mice ( Supplementary Table 2 ). Osteoclast number and perimeter in the vertebrae of FoxO3 C ;LysM-Cre were decreased ( Fig. 3e,f ), as was osteoclast gene expression measured in whole bones ( Supplementary Fig. 4b ), while the expression of bglap was unchanged. FoxOs decrease osteoclast proliferation and lifespan Next, we sought to identify the mechanism by which FoxOs suppress osteoclast numbers. BMMs from FoxO1,3,4 f/f ;LysM-Cre mice formed more osteoclasts when cultured in the presence of M-CSF and RANKL ( Fig. 4a ). This increase was confirmed by the higher mRNA levels of catk, TRAP and calcr ( Fig. 4b ). In addition, when cultured on dentin slices, the area resorbed by the osteoclasts lacking FoxOs was higher, as determined by the lectin-stained pits ( Supplementary Fig. 5a ). The increased osteoclastogenesis was associated with increased proliferation, as determined by cell number ( Supplementary Fig. 5b ) and bromodeoxyuridine (BrdU) staining of macrophages ( Fig. 4c ) but unaltered lifespan of macrophages or osteoclasts ( Supplementary Fig. 5c,d ). Cells from the FoxO3 C ;LysM-Cre mice exhibited the opposite phenotype, including decreased osteoclast formation ( Fig. 4d,e , Supplementary Fig. 5e ), decreased proliferation of macrophages ( Fig. 4f , Supplementary Fig. 5f ), as well as increased osteoclast ( Fig. 4g ), but not macrophage ( Supplementary Fig. 5g ), apoptosis. In line with the role of FoxOs in inhibiting osteoclast progenitor proliferation, the mRNA and protein levels of cyclin D1 were higher in BMMs from FoxO1,3,4 f/f ;LysM-Cre mice ( Fig. 4h,i ). Cells from FoxO3 C ;LysM-Cre mice exhibited opposite changes. 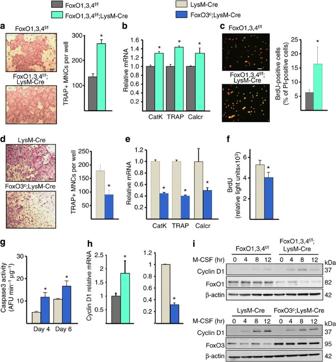Figure 4: FoxOs attenuate osteoclast progenitor proliferation and decrease mature osteoclast lifespan. (a) Representative pictures (left) and number of TRAP-positive multinucleated cells (MNCs) generated from BMMs (right, triplicates). Scale bar, 500 μm. (b) Cathepsin K (CatK), TRAP and calcitonin receptor (calcr) mRNA levels in osteoclast cultures (triplicates). (c) Representative pictures of BrdU (green) and propidium iodide (red) staining (left) and percentage of BrdU-positive cells in BMMs cultures (right; triplicates). Scale bar, 20 μm. (d–f) Same asa–dusing cells from FoxO3C;LysM-Cre and LysM-Cre littermates. (g) Caspase-3 activity in mature osteoclast cultures (triplicates). AFU, arbitrary fluorescent units. (h) Cyclin D1 mRNA and (i) protein levels in BMM cell cultures (triplicate). Bars represent mean and s.d.; *P<0.05 versus respective FoxO1,3,4f/for LysM-Cre cells by Student’st-test. Figure 4: FoxOs attenuate osteoclast progenitor proliferation and decrease mature osteoclast lifespan. ( a ) Representative pictures (left) and number of TRAP-positive multinucleated cells (MNCs) generated from BMMs (right, triplicates). Scale bar, 500 μm. ( b ) Cathepsin K (CatK), TRAP and calcitonin receptor (calcr) mRNA levels in osteoclast cultures (triplicates). ( c ) Representative pictures of BrdU (green) and propidium iodide (red) staining (left) and percentage of BrdU-positive cells in BMMs cultures (right; triplicates). Scale bar, 20 μm. ( d – f ) Same as a – d using cells from FoxO3 C ;LysM-Cre and LysM-Cre littermates. ( g ) Caspase-3 activity in mature osteoclast cultures (triplicates). AFU, arbitrary fluorescent units. ( h ) Cyclin D1 mRNA and ( i ) protein levels in BMM cell cultures (triplicate). Bars represent mean and s.d. ; * P <0.05 versus respective FoxO1,3,4 f/f or LysM-Cre cells by Student’s t- test. Full size image We next investigated whether FoxOs altered the signalling pathways stimulated by M-CSF, including Erk, p38, JNK and Akt. No differences were detected in M-CSF-dependent activation between BMMs from FoxO1,3,4 f/f and FoxO1,3,4 f/f ;LysM-Cre mice, or between BMMs from LysM-Cre and FoxO3 C ;LysM-Cre mice ( Supplementary Fig. 6 ). Stimulations of MAPK, Akt and NF-kB by RANKL were also unaffected by FoxO deletion ( Supplementary Fig. 7 ). Taken together, these findings suggest that FoxOs decrease osteoclast number by attenuating the proliferation of progenitors and decreasing the lifespan of mature osteoclasts. FoxOs stimulate catalase to inhibit H 2 O 2 and bone resorption In view of the antioxidant role of FoxOs in some cell types [20] , [23] , [33] and the present data showing that the levels of catalase decrease along with FoxOs during osteoclast differentiation, we examined whether catalase is indeed a target gene of FoxOs in osteoclasts. Catalase mRNA and protein levels were decreased in BMMs and osteoclasts from FoxO1,3,4 f/f ;LysM-Cre mice and increased in cells from FoxO3 C ;LysM-Cre mice ( Fig. 5a,b ). MnSOD is another FoxO target gene in some cell types. However, in contrast to catalase , MnSOD was not affected by FoxO deletion in osteoclastic cells ( Fig. 5c ). On the basis of the changes in catalase and earlier findings that RANKL increases cellular ROS [12] , [13] , we next examined whether FoxOs altered H 2 O 2 levels in osteoclasts. Cultured osteoclast progenitor cells from FoxO1,3,4 f/f ;LysM-Cre mice exhibited higher H 2 O 2 levels in the absence or in response to RANKL, as compared with cells from control mice ( Fig. 5d ). In contrast, overexpression of FoxO3 prevented the RANKL-induced increase in H 2 O 2 . We have previously shown that low levels of H 2 O 2 prolong mature osteoclast lifespan in cultures from wild-type mice [34] . In the present report we found that low H 2 O 2 levels also increase osteoclast progenitor proliferation. This effect was seen when H 2 O 2 was added to the culture medium ( Supplementary Fig. 8a–c ) or when H 2 O 2 was continuously generated using glucose oxidase ( Supplementary Fig. 8d–g ). Attenuation of H 2 O 2 by adding pegylated catalase to cells from FoxO1,3,4 f/f ;LysM-Cre mice abrogated the high proliferation ( Fig. 5e ) and the elevated cyclin D1 mRNA levels ( Fig. 5f ) in osteoclast progenitors. Moreover, silencing of catalase abrogated the decrease in cyclin D1 mRNA levels in cells from mice overexpressing FoxO3 ( Fig. 5g ). In agreement with these findings, BMMs from catalase knockout mice ( Supplementary Fig. 9a ) had increased ROS ( Supplementary Fig. 9b ) and higher proliferation ( Supplementary Fig. 9c ) than cells from wild-type littermates. 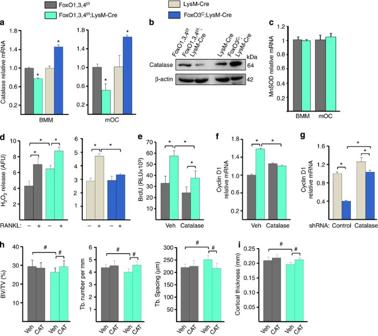Figure 5: FoxOs attenuate bone resorption by decreasing H2O2. (a) Catalase mRNA levels in BMM and in mature osteoclast (mOC) cultures (triplicates). (b) Catalase protein levels in mature osteoclast. (c) MnSOD mRNA (triplicates). (d) H2O2levels using Amplex Red in osteoclast progenitors (triplicates). (e) Proliferation by BrdU labelling; and (f) cyclin D1 mRNA levels in BMM cultures treated with vehicle (veh) or 75 Units ml−1of pegylated catalase (triplicates). (g) Cyclin D1 mRNA levels in BMM silenced for catalase (triplicates). Sh, short hairpin. (h) Four-week-old male mice were administered veh or pegylated catalase (CAT) for 6 weeks. Bone volume relative to the total volume (BV/TV), and trabecular (Tb) number and spacing in vertebrae; and (i) cortical thickness at the midshaft of femur (n=10–11 per group). Bars represent mean and s.d. *P<0.05 by Student’st-test.#P<0.05 by two-way analysis of variance (ANOVA). Figure 5: FoxOs attenuate bone resorption by decreasing H 2 O 2 . ( a ) Catalase mRNA levels in BMM and in mature osteoclast (mOC) cultures (triplicates). ( b ) Catalase protein levels in mature osteoclast. ( c ) MnSOD mRNA (triplicates). ( d ) H 2 O 2 levels using Amplex Red in osteoclast progenitors (triplicates). ( e ) Proliferation by BrdU labelling; and ( f ) cyclin D1 mRNA levels in BMM cultures treated with vehicle (veh) or 75 Units ml −1 of pegylated catalase (triplicates). ( g ) Cyclin D1 mRNA levels in BMM silenced for catalase (triplicates). Sh, short hairpin. ( h ) Four-week-old male mice were administered veh or pegylated catalase (CAT) for 6 weeks. Bone volume relative to the total volume (BV/TV), and trabecular (Tb) number and spacing in vertebrae; and ( i ) cortical thickness at the midshaft of femur ( n =10–11 per group). Bars represent mean and s.d. * P <0.05 by Student’s t -test. # P <0.05 by two-way analysis of variance (ANOVA). Full size image To determine whether the low bone mass of the FoxO1,3,4 f/f ;LysM-Cre mice was because of increased H 2 O 2 in osteoclasts, we administered pegylated catalase to 4-week-old FoxO1,3,4 f/f ;LysM-Cre mice for 28 days. Catalase had no effect on the bone mass of the control littermate mice but it rescued the low bone mass phenotype of the FoxO1,3,4 f/f ;LysM-Cre mice ( Fig. 5h ). Specifically, catalase abrogated the decrease in cancellous BMD, bone volume and trabecular number, as well as the increase in trabecular spacing. Catalase also prevented the low cortical bone thickness of the FoxO1,3,4 f/f ;LysM-Cre mice ( Fig. 5i ). Similar results were obtained when we administered the unspecific antioxidant NAC to 4-week-old FoxO1,3,4 f/f ;LysM-Cre mice for 6 weeks ( Supplementary Fig. 10 ). Taken together, these results indicate that FoxOs decrease osteoclast numbers and bone resorption by lowering H 2 O 2 levels because of an increase in catalase. Mitochondrial H 2 O 2 in osteoclasts stimulates bone resorption We sought independent confirmation for the role of H 2 O 2 in cells of the osteoclast lineage using mice in which we overexpressed mitochondria-targeted catalase specifically in osteoclasts by crossing mice with a conditionally activated catalase transgene targeted to the mitochondria (MitoCat) [35] with LysM-Cre mice. The MitoCat transgene caused a threefold increase in catalase activity in osteoclasts from the MitoCat;LysM-Cre mice as compared with LysM-Cre littermates ( Fig. 6a ). Catalase activity was unaltered in the kidney, brain and liver of MitoCat;LysM-Cre mice, confirming the specificity of the targeted expression. 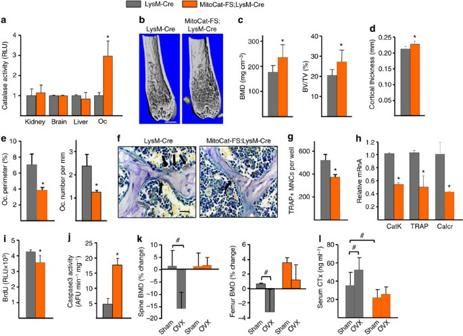Figure 6: Mitochondria-derived H2O2promotes osteoclast generation and bone resorption. (a) Catalase activity in soft tissues and osteoclast (Oc) cultures from LysM-Cre (n=4) and MitoCat-FS;LysM-Cre (n=4) littermates. RLU, relative light units. (b) Representative μCT images of distal femur of 12-week-old male mice. Scale bar, 1 mm. (c) Cancellous BMD and bone volume relative to the total volume (BV/TV) of 12-week-old male LysM-Cre (n=12) and MitoCat-FS;LysM-Cre (n=10) littermates. (d) Cortical thickness determined by μCT in femoral diaphysis of the samples described inc. (e) Osteoclasts in cancellous bone of vertebra from mice described inc(n=6 mice per group). (f) Histological sections of bones, described ine, stained for TRAP activity (osteoclasts stain red). Scale bar, 20 μm. (g) Number of TRAP-positive MNCs generated from BMMs (triplicates). (h) Cathepsin K (CatK), TRAP and calcitonin receptor (calcr) mRNA levels in osteoclast cultures (triplicates). (i) Proliferation by BrdU labelling in BMM cultures (triplicates). (j) Caspase-3 activity in mature osteoclast cultures (triplicates). AFU, arbitrary fluorescent units. (k) Twelve-week-old mice were sham-operated or OVX and killed 6 weeks later. BMD by DEXA as % change from the initial BMD in LysM-Cre sham (n=10), LysM-Cre OVX (n=9), MitoCat-FS;LysM-Cre sham (n=7) and MitoCat-FS;LysM-Cre OVX (n=7) mice. (l) Serum concentration of a collagen degradation product (CTx), in mice described ink, at the time of killing. Bars represent mean and s.d. *P<0.05 by Student’st-test.#P<0.05 by two-way ANOVA. Figure 6: Mitochondria-derived H 2 O 2 promotes osteoclast generation and bone resorption. ( a ) Catalase activity in soft tissues and osteoclast (Oc) cultures from LysM-Cre ( n =4) and MitoCat-FS;LysM-Cre ( n =4) littermates. RLU, relative light units. ( b ) Representative μCT images of distal femur of 12-week-old male mice. Scale bar, 1 mm. ( c ) Cancellous BMD and bone volume relative to the total volume (BV/TV) of 12-week-old male LysM-Cre ( n =12) and MitoCat-FS;LysM-Cre ( n =10) littermates. ( d ) Cortical thickness determined by μCT in femoral diaphysis of the samples described in c . ( e ) Osteoclasts in cancellous bone of vertebra from mice described in c ( n =6 mice per group). ( f ) Histological sections of bones, described in e , stained for TRAP activity (osteoclasts stain red). Scale bar, 20 μm. ( g ) Number of TRAP-positive MNCs generated from BMMs (triplicates). ( h ) Cathepsin K (CatK), TRAP and calcitonin receptor (calcr) mRNA levels in osteoclast cultures (triplicates). ( i ) Proliferation by BrdU labelling in BMM cultures (triplicates). ( j ) Caspase-3 activity in mature osteoclast cultures (triplicates). AFU, arbitrary fluorescent units. ( k ) Twelve-week-old mice were sham-operated or OVX and killed 6 weeks later. BMD by DEXA as % change from the initial BMD in LysM-Cre sham ( n =10), LysM-Cre OVX ( n =9), MitoCat-FS;LysM-Cre sham ( n =7) and MitoCat-FS;LysM-Cre OVX ( n =7) mice. ( l ) Serum concentration of a collagen degradation product (CTx), in mice described in k , at the time of killing. Bars represent mean and s.d. * P <0.05 by Student’s t -test. # P <0.05 by two-way ANOVA. Full size image MitoCat;LysM-Cre mice had higher cancellous BMD and bone volume in the femur at 12 ( Fig. 6b,c ) and 24 weeks ( Supplementary Table 3 ). A similar increase in cancellous bone volume was seen in the vertebrae ( Supplementary Table 3 ). Cortical thickness was also increased in these mice ( Fig. 6d ) as a result of reduced endosteal perimeter ( Supplementary Table 3 ), suggesting decreased endocortical resorption. Consistent with the higher bone mass, MitoCat;LysM-Cre mice had decreased osteoclast perimeter and number per cancellous bone surface ( Fig. 6e,f ). Similar to the case with cells from mice overexpressing FoxO3, ex vivo cultures of bone marrow cells from MitoCat;LysM-Cre mice formed fewer osteoclasts ( Fig. 6g,h ). In addition, macrophages from MitoCat;LysM-Cre exhibited decreased proliferation ( Fig. 6i ) and mature osteoclasts displayed increased apoptosis ( Fig. 6j ). Finally, to examine the importance of osteoclast H 2 O 2 during pathologic bone resorption, we performed ovariectomy (OVX) of MitoCat;LysM-Cre and LysM-Cre littermates at 3 months of age, and examined the impact on bone mass 6 weeks later. OVX caused the expected decrease of BMD in the spine and femur of LysM-Cre control mice ( Fig. 6k ). In contrast, MitoCat;LysM-Cre littermate mice were protected from the OVX-induced bone loss. Consistent with the bone changes, osteoclast resorption markers in the serum were increased with OVX in the control mice but were unchanged in MitoCat;LysM-Cre mice ( Fig. 6l ), demonstrating that the OVX-induced increase in bone resorption was prevented by the MitoCat transgene. These results indicate that elevated H 2 O 2 production in the mitochondria of osteoclasts is a seminal culprit of the increased bone resorption caused by loss of oestrogens. Generation of oxygen-derived free radicals is an inescapable consequence of aerobic metabolism and occurs primarily in mitochondria because of the escape of electrons passing through the electron transport chain [36] , [37] . This process generates superoxide, which is highly reactive and short-lived. Superoxide is rapidly converted to the more stable and less reactive H 2 O 2 , the most abundant form of ROS that diffuses freely through the mitochondrial membranes into the cytosol [19] , [38] , [39] . These and other ROS can cause harm by damaging proteins, lipids and DNA leading to cell demise and have, therefore, been implicated in the biology of aging and aging-related diseases for over 60 years [40] . ROS, however, also function as propagators of intracellular signalling for physiological cell function [41] , [42] , [43] . These seemingly different actions may depend on the levels of ROS generated during signalling (lower) as opposed to stress (higher), and perhaps fundamentally different ways by which different cell types handle or compartmentalize ROS [36] , [44] . In the work presented here, we have elucidated that M-CSF and RANKL promote the accumulation of H 2 O 2 in osteoclasts and their progenitors via an Akt-mediated repression of FoxO transcription that lowers catalase protein levels. H 2 O 2 , in turn, stimulates osteoclast progenitor proliferation and prolongs the lifespan of mature osteoclasts ( Fig. 7 ). To the best of our knowledge, this is the first paradigm that pro-differentiating factors repress FoxOs to allow the accumulation of ROS for signalling. In support of a critical and cell-autonomous role of FoxOs in the regulation of osteoclast number and the volume of bone mass, we found that mice with loss or gain of FoxO function in osteoclasts have diametrically opposite skeletal phenotypes: increased versus decreased osteoclast number and lower versus higher bone mass, respectively. In addition, we have established that the effects of FoxOs on the bone are the result of H 2 O 2 changes. We did so by demonstrating that the consequences of the loss of FoxO function on osteoclast number and bone resorption were prevented by the systemic administration of catalase. Conversely, the changes caused by gain of FoxO3 function were simulated by the osteoclast-specific expression of mitochondria-targeted catalase. Hence, increased ROS levels, and in particular elevation of H 2 O 2 , is a critical and regulated step of osteoclastogenesis and thus bone resorption—not a mere epiphenomenon of increased mitochondria number and/or function required to meet the high energy demands of osteoclastic bone resorption. 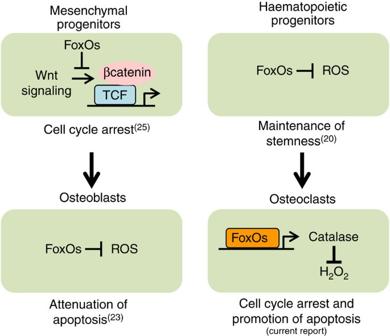Figure 7: Effects of FoxOs on the birth and death of osteoblasts and osteoclasts. Aberrant cell number is the culprit of most metabolic bone diseases, including osteoporosis3. Earlier work, with targeted loss or gain of FoxO function at different stages of osteoblast differentiation in mice, revealed a restraining effect of FoxOs on Wnt signalling in mesenchymal progenitors. This effect leads to a decrease in the number of osteoblasts and is independent of the antioxidant properties of FoxOs. On the other hand, FoxOs promote the survival of mature osteoblasts. Previous work has also elucidated that FoxOs reduce ROS and promote stemness in haematopoietic stem cells. The present report shows that FoxOs prevent the accumulation of H2O2in osteoclasts and their progenitors by increasing the expression of catalase and, thereby, promote cell cycle arrest and apoptosis. Figure 7: Effects of FoxOs on the birth and death of osteoblasts and osteoclasts. Aberrant cell number is the culprit of most metabolic bone diseases, including osteoporosis [3] . Earlier work, with targeted loss or gain of FoxO function at different stages of osteoblast differentiation in mice, revealed a restraining effect of FoxOs on Wnt signalling in mesenchymal progenitors. This effect leads to a decrease in the number of osteoblasts and is independent of the antioxidant properties of FoxOs. On the other hand, FoxOs promote the survival of mature osteoblasts. Previous work has also elucidated that FoxOs reduce ROS and promote stemness in haematopoietic stem cells. The present report shows that FoxOs prevent the accumulation of H 2 O 2 in osteoclasts and their progenitors by increasing the expression of catalase and, thereby, promote cell cycle arrest and apoptosis. Full size image Our in vitro work, using cells in which catalase was knocked down, suggest that this enzyme is critical for the attenuation of osteoclast progenitor proliferation by FoxOs. However, it remains possible that in addition to catalase, which localizes to the peroxisomes, FoxOs attenuate H 2 O 2 accumulation via other mechanisms, such as, for example, stimulation of expression of cytoplasmic peroxiredoxins. A requirement of ROS signalling in cell differentiation and function has been shown earlier in vitro —for example, in the case of adipocyte differentiation [45] and insulin secretion by β cells [46] . In addition, there is genetic evidence that signalling ROS promote longevity in yeast and Caenorhabditis elegans [47] , [48] , [49] , [50] , and that ROS are involved in angiotensin II signal propagation [35] and immunoregulation [51] , [52] in mammals, but only under pathologic conditions. The elucidation of the role of mitochondria-derived H 2 O 2 in osteoclastogenesis and the maintenance of bone mass in the present report represents the first functional demonstration of the role of signalling ROS in mammalian physiology. Elucidation of the specific molecular targets of H 2 O 2 in osteoclast differentiation and bone mass maintenance will require future studies. In addition to mitochondria, ROS, including H 2 O 2 , are generated at the plasma membrane by the NADPH oxidases Nox1 and Nox2 (ref. 53 ). In vitro studies have suggested that ROS produced by Nox1 and Nox2 may participate in osteoclast differentiation triggered by RANKL signalling [13] . The fact that the loss of FoxO function or the targeting of catalase to mitochondria in osteoclasts attenuated, but did not abolish, osteoclastogenesis and bone resorption suggests that besides FoxO downregulation, other mechanisms contribute to H 2 O 2 accumulation during osteoclast differentiation. Nonetheless, H 2 O 2 and perhaps other ROS accumulation is most likely indispensable for the transition of osteoclast progenitors to mature osteoclasts, as evidenced by the finding that antioxidants completely prevent osteoclast generation in vitro [13] , [17] . Earlier work of ours with targeted loss or gain of FoxO function at different stages of osteoblast differentiation in mice revealed a restraining effect of FoxOs on Wnt signalling in lineage-committed osteoblast progenitors [25] ( Fig. 7 ). This effect leads to a decrease in the number of matrix-synthesizing osteoblasts and bone mass. Unlike the effects of FoxOs on osteoclasts, the effect on the committed osteoblast progenitors is independent of the antioxidant properties of FoxOs. On the other hand, FoxOs promote the survival of mature osteoblasts and osteocytes as a result of ROS attenuation and they may also promote the maintenance of self-renewing mesenchymal stem cells by such antioxidant actions [20] , [54] , [55] . On the basis of this evidence, we proposed recently that the overriding function of FoxOs in osteoblasts is to provide an optimal balance among the maintenance of self-renewing stem cells, the replication of lineage-committed intermediates and the survival of the terminally differentiated osteoblast progeny, most likely for the purpose of compensatory adaptations to stresses that accumulate in bone with advancing age [25] . Nonetheless, as is the case with several other defense responses against aging [56] , FoxO activation by cellular stressors accumulating with age may eventually aggravate the effects of aging on bone and become a pathogenetic mechanism of involutional osteoporosis. The results of the present work showing that an increase in H 2 O 2 production in osteoclasts promotes osteoclastogenesis and stimulates bone resorption, taken together with our earlier findings that an increase in ROS promotes osteoblast and osteocyte apoptosis [23] , indicate that there are fundamental differences in the way osteoblasts and osteoclasts handle ROS. Thus, increased ROS generation by dysfunctional mitochondria with age may be a seminal molecular mechanism of the progressive imbalance between bone resorption and formation that is the hallmark of skeletal involution. The loss of bone caused by oestrogen deficiency in animals and humans is associated with an increase in osteoclastogenesis, increased osteoclast numbers and increased resorption [3] , [57] . In addition, we and others have shown earlier that similar to aging, oestrogen loss in mice increases the generation of ROS and systemic administration of antioxidants attenuates the loss of bone mass caused by the loss of oestrogens [17] , [34] . On the basis of this and evidence that oestrogens stimulate antioxidant mechanisms in osteoclasts, we and others have suggested earlier that attenuation of ROS by oestrogens contribute to their bone-protective effects [16] . However, it remains unclear whether the antioxidant effects of oestrogens result from direct actions on osteoclasts or indirect actions mediated by osteoblast progenitors or B lymphocytes [58] , [59] , [60] , [61] . Our findings that mice with mitochondria-targeted catalase in osteoclasts are protected from the loss of bone caused by oestrogen deficiency strongly suggests that mitochondria-derived H 2 O 2 is indeed the culprit of the pathologic bone resorption that ensues upon loss of oestrogens. Similar to oestrogen deficiency, an increase in ROS has been implicated in the increased bone resorption caused by inflammatory arthritis and iron overload [18] , [62] , [63] . In closing, the work presented here reveals that H 2 O 2 accumulation in response to M-CSF and RANKL (via an Akt/FoxO cascade) is a critical control node of osteoclastogenesis and bone resorption, under both physiologic and pathologic conditions. Therefore, decreasing H 2 O 2 production in mitochondria may be a rational pharmacotherapeutic approach to the treatment of diseases associated with high bone resorption, including postmenopausal osteoporosis, arthritis and iron overload. Targeted FoxO activation in osteoclastic cells could be one mechanistic approach for achieving this goal. Notably, decreasing H 2 O 2 production by targeted expression of catalase to mitochondria in mice also prevents the age-associated energy imbalance, muscle insulin resistance [64] , hypertensive cardiomyopathy and pressure overload-induced heart failure [35] , beta amyloid toxicity [65] and hearing loss [66] . Hence, cell-specific antioxidants or antioxidants targeted to specific subcellular compartments could simultaneously combat osteoporosis and other degenerative disorders resulting from shared mechanisms of aging. Animal experimentation We generated loss of FoxO function experimental mice by a two-step breeding strategy. Homozygous LysM-Cre mice (C57BL/6) were crossed with FoxO1,3,4 f/f mice (mixture of FVBn and 129Sv) [67] to generate mice that were heterozygous for FoxO1, 3 and 4 conditional alleles with and without the Cre allele. The FoxO1,3,4 f/+ ;LysM-Cre were backcrossed with the FoxO1,3,4 f/f mice for two successive generations to obtain the experimental FoxO1,3,4 f/f ;LysM-Cre mice and the FoxO1,3,4 f/f control littermates. For subsequent studies, we intercrossed the FoxO1,3,4 f/f mice with and without the Cre alleles. Genotypes of the offspring were determined by PCR using primers specific for LysM-Cre 5′-CCCAGAAATGCCAGATTACG-3′ mutant (bp 700), 5′-CTTGGGCTGCCAGAATTTCTC-3′ common (bp 700 and 350) and 5′-TTACAGTCGCCAGGCTGAC-3′ wild-type (bp 350); and that detect the wild-type and floxed Foxo1, 3 and 4 alleles [67] . We generated gain of FoxO function experimental mice by crossing homozygous LysM-Cre mice with hemizygous FoxO3 C mice (C57BL/6) [23] to generate offsprings that were all hemizygous for the LysM-Cre transgene with or without the FoxO3 C transgene. Transgenic offsprings were identified with PCR using the following primer sequences: mutant (101 bp) 5′-GAGTCGCTCGGTACGATTTA-3′ reverse (101 bp) 5′-CGGGAGGCTAGCATAATCAG-3′. We generated experimental mice with human catalase targeted to the mitochondria by crossing homozygous LysM-Cre mice with hemizygous MitoCat-FS mice (C57BL/6) [35] to generate offspring that were all hemizygous for the LysM-Cre transgene and 50% of these were also hemizygous for the MitoCat-FS transgene. Transgenic offsprings were identified with PCR using the following primer sequences: MitoCat forward 5′-CTGAGGATCCTGTTAAACAATGC-3′ MitoCat reverse 5′-CTATCTGTTCAACCTCAGCAAAG-3′, product size 1,087 bp. We injected 4-week-old FoxO1,3,4 f/f ;LysM-Cre and FoxO1,3,4 f/f littermate mice daily with 200 μg g −1 pegylated catalase (Sigma-Aldrich, St. Louis, MO, USA) or vehicle (phosphate-buffered saline) for 28 days. In a second experiment, we injected 4-week-old FoxO1,3,4 f/f ;LysM-Cre and FoxO1,3,4 f/f littermate mice daily with 100 mg kg −1 body weight NAC (Sigma-Aldrich) or saline, for 6 weeks. We ovariectomized or sham-operated 12-week-old MitoCat-FS;LysM-Cre and LysM-Cre littermates that were stratified by the presurgical spinal BMD measurement. After 6 weeks, we measured BMD, killed the animals and dissected the tissues for further analyses. Protocols involving genetically modified mice and their wild-type littermates were approved by the Institutional Animal Care and Use Committees of the University of Arkansas for Medical Sciences and the Central Arkansas Veterans Healthcare System. BMD determination We determined BMD using a PIXImus densitometer (GE-Lunar Corp.) running software version 2.0. The spine window was a rectangle depending on animal body length, reaching from just below the skull to the base of the tail. The femoral window captured the right femur. Scan acquisition time was 4 min and analysis time was 6 min. We sedated the mice with isoflurane during scanning to keep the animals motionless for the required 4 min and to facilitate rapid post-examination recovery. We monitored the animals by observation of the righting reflex, respiration and heart rate. In experiments in which mice were administered antioxidants or were ovariectomized, we used initial spinal BMD determinations to randomly allocate animals to treatment groups with equivalent BMD values. Micro-CT analysis We dissected the femur and vertebrae (L4 or L5), cleaned them of soft tissues, fixed them in 10% Millonig’s formalin and gradually dehydrated them into 100% ethanol. We loaded bones into 12.3-mm diameter scanning tubes and imaged them in a μCT (model μCT40, Scanco Medical). We integrated the scans into three-dimensional (3D) voxel images (1,024 × 1,024 pixel matrices for each individual planar stack) and used a Gaussian filter (sigma=0.8, support=1) to reduce signal noise. We applied a threshold of 200 to all scans, at medium resolution ( E =55 kVp, I =145 μA, integration time=200 ms). We scanned whole vertebra with a transverse orientation excluding any bone outside the vertebral body. We manually excluded the cortical bone and the primary spongiosa from the analysis. In the distal femur, 151 transverse slices were taken from the epicondyles and extending towards the proximal end of the femur. The cortical bone and the primary spongiosa were manually excluded from the analysis. All trabecular measurements were made by drawing contours every 10–20 slices and using voxel counting for bone volume per tissue volume and sphere-filling distance transformation indices, without pre-assumptions about the bone shape as a rod or plate for trabecular microarchitecture. We measured cortical thickness at the femoral mid-diaphysis. Image-processing language scripts including the ‘cl image’ command were used to obtain the femoral endosteal and periosteal perimeters. Histomorphometry We fixed the lumbar vertebrae (L2–L4) for 24 h in 10% Millonig’s formalin and decalcified in 14% EDTA for 1 week. Vertebrae were then embedded in paraffin, and 5-μm longitudinal sections were obtained. After de-paraffinization and rehydration, sections were incubated with 0.2 M acetate buffer containing 10% (vol/vol) naphthol-AS-BI-phosphate at 37 °C for 30 min. The sections were then incubated with pararosaniline chloride (1.5 g ml −1 ) for 5 min and counterstained with 0.1% fast green. In some experiments (indicated in the text), we embedded undecalcified vertebrae in methyl methacrylate and 4- to 8-μm longitudinal sections were obtained. Before staining, we eluted the plastic with 2-methoxyethyl acetate. Decalcified and undecalcified TRAP-stained sections, counterstained with toluidine blue, were used for osteoclast enumeration. Osteoclast counts were performed using a computer and digitizer tablet (OsteoMetrics) interfaced to a Zeiss Axioscope (Carl Zeiss) with a drawing tube attachment. The numbers of TRAP-positive multinucleated cells on the cancellous perimeter (osteoclast number) were measured directly. Terminology recommended by the Histomorphometry Nomenclature Committee of the American Society for Bone and Mineral Research was used in this study [68] . Cell culture We obtained bone marrow cells by flushing the tibiae and femurs from 2- to 3-month-old mice with α-MEM medium (Invitrogen). After the red blood cells were removed with ACK buffer (0.01 mM EDTA, 0.011 M KHCO 3 and 0.155 M NH 4 Cl, pH 7.3), we suspended the cells in α-MEM complete media containing 10% (v/v) fetal bovine serum, 100 U ml −1 penicillin and 100 μg ml −1 streptomycin and incubated the cells for 24 h in the presence of 10 ng ml −1 M-CSF. We collected the non-adherent cells and cultured with 30 ng ml −1 M-CSF for 3 days to generate bone marrow-derived macrophages. To generate pre-osteoclasts and osteoclasts we cultured bone marrow-derived macrophages (50,000 cells cm −2 ) with 30 ng ml −1 M-CSF and 30 ng ml −1 RANKL (R&D Systems) for 2 and 4 days, respectively, in α-MEM complete media. We fixed the pre-osteoclast and osteoclast cultures with 10% neutral buffered formalin for 15 min and stained for TRAP using the Leukocyte Acid Phosphatase Assay Kit, following the manufacturer’s instructions (Sigma-Aldrich). A pre-osteoclast was defined as a round mononuclear TRAP-positive cell and an osteoclast as a multinuclear TRAP-positive cell. We quantified intracellular ROS using dichlorodihydrofluorescein dye [69] and H 2 O 2 using the Amplex Red Assay Kit (Invitrogen). We measure catalase activity using the OxiSelect Catalase Activity Assay Kit, following the manufacturer’s instructions (Cell Biolabs). For all assays we plated cells in triplicate. Caspase-3 activity We lysed the cells in 20 mM Tris-HCl (pH 7.5), 150 mM NaCl, 1 mM EDTA, 10 mM NaF, 1 mM sodium orthovanadate, 5 mg ml −1 leupeptin, 0.14 U ml −1 aprotinin, 1 mM phenylmethylsulfonylfluoride and 1% Triton X-100. Lysates (100 mg protein) were incubated with 50 mM DEVD-AFC in 50 mM HEPES (pH 7.4), 100 mM NaCl, 0.1% CHAPS, 10 mM dithiothreitol, 1 mM EDTA and 10% glycerol. Caspase-3 activity was measured by determining the degradation of the fluorometric substrate DEVD-AFC. We measured the released fluorescent in a microplate fluorescence reader with excitation/emission wavelengths of 340/542 nm. We measured protein concentration using a Bio-Rad detergent-compatible kit (Bio-Rad). Cell proliferation assay We cultured BMMs for 2–4 days with 30 ng ml −1 M-CSF. We fixed the cells in 1% (w/v) paraformaldehyde (Sigma) on ice for 15 min, and then stained in Alexa Fluor 488 dye-labelled anti-BrdU antibody (Invitrogen) for 30 min at room temperature. To determine the total cellular DNA content, we stained BMMs in propidium iodide for an additional 30 min at room temperature. We confirmed each labelling using fluorescence microscopy. We determined the percentage of BrdU-positive cells by counting the number of BrdU-positive above propidium iodide-positive cells. We also assayed proliferation by BrdU incorporation with a kit from Roche Diagnostics following the manufacturer’s instructions. Transient transfections and luciferase assay We cultured cells on 48-well plates and 16 h later transfected cells with 0.2 μg of a reporter plasmid containing six copies of daf-16 family protein-binding element (FoxO-luc), 0.01 μg of Renilla (control reporter) and 0.2 μg of pcDNA or 0.2 μg of FoxO1, FoxO3 or FoxO4 expression plasmids using Lipofectamine Plus (Invitrogen). Twenty-four hours later we treated cells with or without RANKL for 16 h. We determined luciferase activity using the Dual-LuciferaseReporter assay system (Promega), according to the manufacturer’s instructions. We measured light intensity with a luminometer and divided luciferase activity by the control reporter to normalize for transfection efficiency. RNA isolation and quantitative RT–PCR analysis We dissected soft tissues and bones that were frozen immediately upon harvest from mice. We extracted the total RNA from tissues and cultured cells using Ultraspec (Biotecx Laboratories) and reverse-transcribed the RNA using the High-Capacity cDNA Archive Kit (Applied Biosystems) according to the manufacturer’s instructions. Primers and probes for the different genes were manufactured by the TaqMan Gene Expression Assays service (Applied Biosystems). We carried out qRT–PCR using the following Taqman assays: RANKL (Mm0041908_m1); cathepsin K (Mm01255862_g1); TRAP (Mm00475698_m1); calcitonin receptor (Mm0043221_m1); catalase (Mm00437992_m1); MnSOD (Mm00449726_m1); FoxO1 (Mm00490672_m1); FoxO3 (Mm00490673_m1); FoxO4 (Mm00840140_g1); Cyclin D1 (Mm00432359_m1). Primers and probe for HA-FoxO3 and OCN were manufactured by the Assays-on-demand service (Applied Biosystems): 5′-CTCTGACTGACCGCGTTACTC-3′ and 5′-GCCAAAATGATGAGACAGCACAATA-3′; 5′-GCTGCGCTCTGTCTCTCTGA-3′ and 5′-TGCTTGGACATGAAGGCTTTG-3′. The mRNA levels were calculated by normalizing to the house-keeping gene ribosomal protein S2 (Mm00475528_m1) using the Δ C t method [70] . Western blot We obtained nuclear extracts using the Nuclear Extract Kit (Active Motif) according to the manufacturer’s instructions. We determined FoxO1, 3 and 4 levels in cultured cell lysates using a rabbit monoclonal antibody for FoxO1 (Cell Signalling no. 2880, 1:1,000), a rabbit monoclonal antibody for FoxO3 (Cell Signalling no. 9467, 1:1,000) and a rabbit polyclonal antibody for FoxO4 (Cell Signalling no. 9472, 1:1,000). We analysed protein levels of HA-FoxO3 or β-actin using mouse monoclonal antibodies (Cell Signalling no. 2367, 1:1,000 and Sigma sc-81178, 1:2,000, respectively). We determined protein levels of catalase using a rabbit polyclonal antibody (Santa Cruz Biotechnology sc-50508, 1:500). We determined MAPKs and Akt levels in cell lysates using mouse monoclonal antibodies for p-Erk (Santa Cruz Biotechnology sc-7383, 1:500) and p-Jnk (Cell Signalling no. 9255, 1:1,000), rabbit monoclonal antibodies for p-p38 (Cell Signalling no. 9215, 1:1,000) and p-Akt (Cell Signalling no. 4058, 1:1,000), rabbit polyclonal antibodies for Erk (Santa Cruz Biotechnology sc-94, 1:500), p38 (Cell Signalling no. 9212, 1:1,000) and Akt (Cell Signalling no. 9272, 1:1,000) and a mouse monoclonal antibody for Jnk (Santa Cruz Biotechnology sc-1648, 1:500). We analysed the phosphorylation levels of FoxO1 (no. 9461, 1:1,000), FoxO3/FoxO1 (no. 9464, 1:1,000) and GSK3β (no. 9336, 1:1,000) using rabbit polyclonal antibodies (Cell Signalling). We determined cyclin D1 levels in cell lysates using rabbit polyclonal antibody (Santa Cruz Biotechnology sc-753, 1:500). Full size blots can be found in Supplementary Fig. 11 . Quantification of the intensity of the bands in the autoradiograms was performed using a VersaDocTM imaging system (Bio-Rad). Lentiviral particle transduction We used a catalase short hairpin RNA lentiviral infection system (Santa Cruz Biotechnology) according to the manufacturer’s instructions. In brief, we incubated bone marrow-derived macrophages for 10–12 h with the lentiviral particles (10 μl per well in six-well plate) in the presence of 30 ng ml −1 M-CSF and 5 μg ml −1 polybrene (Santa Cruz Biotechnology). Non-targeted shRNA lentiviral particles (Santa Cruz Biotechnology) were used as a scrambled shRNA sequence control. We further cultured the infected cells with M-CSF for 24 h and then incubated with 1 μg ml −1 puromycin (Santa Cruz Biotechnology) for 72 h to remove uninfected cells. Statistics We used two-way analysis of variance or Student’s t -test to detect significant treatment effects, after determining that the data were normally distributed and exhibited equivalent variances. All t -tests were two-sided. We used Bonferroni corrections for multiple comparisons. We considered P -values <0.05 as significant. Error bars in all figures represent s.d. How to cite this article: Bartell, S. M. et al. FoxO proteins restrain osteoclastogenesis and bone resorption by attenuating H 2 O 2 accumulation. Nat. Commun. 5:3773 doi: 10.1038/ncomms4773 (2014).